Reduced plumage and flight ability of a new Jurassic paravian theropod from China Recent discoveries of feathered theropod dinosaurs in the Middle-Late Jurassic Tiaojishan Formation of western Liaoning Province, north-eastern China, have considerably challenged our understanding of the evolution and biology of the Paraves (the most-inclusive clade containing Passer domesticus Linnaeus, 1758 but not Oviraptor philoceratops Osborn, 1924; see Supplementary information ) [1] , [2] , [3] . Large pennaceous feathers were already developed on the tail, forelimbs and hindlimbs, and particularly on the metatarsus and pes, of the troodontid Anchiornis [2] . It has been postulated that large pennaceous feathers first evolved distally on the hindlimbs, as on the forelimbs and tail, in basal paravian theropods and only spread proximally at a subsequent stage in theropod evolution [2] . Moreover, the organization of the pedal feathers into a coherent planar surface suggests that they potentially had some aerodynamic function in Anchiornis [2] . And adding the new taxa Xiaotingia and Anchiornis from the Tiaojishan Formation in a phylogenetic analysis of paravian theropods challenges the pivotal position of the iconic Archaeopteryx , regarded from its discovery as the most primitive bird, shifting it to the Deinonychosauria (the most-inclusive clade containing Dromaeosaurus albertensis Matthew and Brown, 1922 but not P. domesticus Linnaeus, 1758; see Supplementary information ) [3] . Here we describe a new troodontid theropod from the Tiaojishan Formation of western Liaoning Province. Although it resembles Anchiornis from an osteological point of view, this new troodontid is characterized by a reduced plumage, in comparison with other Middle-Late Jurassic feathered deinonychosaurians: large pennaceous feathers are absent from its tail, metatarsus and pes. The plumage of paravian theropods was already diversified by the Late Jurassic, obviously adapted to different ecological niches. Systematic palaeontology Class Theropoda Marsh, 1881 Order Maniraptora Gauthier, 1986 Suborder Troodontidae Gilmore, 1924 Eosinopteryx brevipenna gen. et sp. nov. Etymology Eo , Greek for daybreak, dawn; sino , Latin for Chinese; pteryx , Greek for feather, wing; brevi , Latin for short; penna , Latin for feather. Holotype YFGP (Yizhou Fossil & Geology Park)-T5197, a complete articulated skeleton with associated integumentary structures ( Fig. 1 ; see Methods for provenance and authenticity of the holotype specimen). 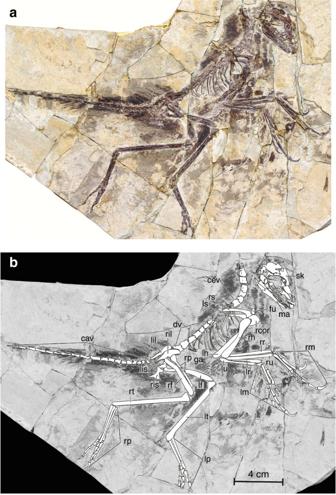Figure 1:Eosipnopteryx brevipennaYFGP-T5197. (a) Photograph and (b) line drawing. cav, caudal vertebrae, cev, cervical vertebrae; dv, dorsal vertebrae; fu, furcula; ga, gastralia; lf, left femur; lh, left humerus; lil, left ilium; lis, left ischium; lm, left manus, lp, left pes; lr, left radius; ls, left scapula; lt, left tibia; lu, left ulna; ma, mandible; rcor, right coracoid; rf, right femur; rh, right humerus; ril, right ilium; ris, right ischium; rm, right manus; rp, right pes; rr, right radius, rs, right scapula; rt, right tibia; ru, right ulna; sk, skull. Figure 1: Eosipnopteryx brevipenna YFGP-T5197. ( a ) Photograph and ( b ) line drawing. cav, caudal vertebrae, cev, cervical vertebrae; dv, dorsal vertebrae; fu, furcula; ga, gastralia; lf, left femur; lh, left humerus; lil, left ilium; lis, left ischium; lm, left manus, lp, left pes; lr, left radius; ls, left scapula; lt, left tibia; lu, left ulna; ma, mandible; rcor, right coracoid; rf, right femur; rh, right humerus; ril, right ilium; ris, right ischium; rm, right manus; rp, right pes; rr, right radius, rs, right scapula; rt, right tibia; ru, right ulna; sk, skull. Full size image Locality and horizon Yaolugou, Jianchang, western Liaoning, China; Middle-Late Jurassic Tiaojishan Formation [1] , [2] , [3] . Diagnosis A small paravian maniraptoran theropod that possesses the following osteological autapomorphies: a short snout, about 82% the length of the orbit; a lacrimal with a long posterior process participating in about half the length of the dorsal margin of the orbit and a vestigial anterior process; a short tail, composed of 20 caudal vertebrae, 2.7 times the length of the femur; chevrons reduced to small rod-like elements below the proximal 8th or 9th caudal; an ilium with a proportionally long, low and distally tapering postacetabular process (ratio ‘length/height at mid-length’=5), and pedal unguals shorter than corresponding penultimate phalanges. The plumage of this taxon is characterized by the absence of rectrices (versus other paravians with preserved plumage) and feathers on metatarsus and pes (versus other troodontids with preserved plumage on the hindlimb). Description The holotype of E. brevipenna is small, just 30 cm long ( Fig. 1 ). The skull has a subtriangular lateral profile produced by a shallow snout and expanded postorbital region ( Fig. 2 ). Unlike Anchiornis [2] , the snout of Eosinopteryx is distinctly shorter (about 82% of orbital length) than its orbit. Both the rostral plate and the maxillary process of the premaxilla are particularly short. The posterior process of the lacrimal is elongated and straight, participating in about half the length of the dorsal margin of the orbit, whereas the anterior process is vestigial. The postorbital process of the jugal is broader than in Anchiornis [2] , whereas the triradiate postorbital is larger than in Archaeopteryx [4] and forms a complete postorbital bar with the jugal. There is no trace of a mandibular fenestra. The dentary has a groove that widens posteriorly and contains a row of foramina as in Archaeopteryx , Anchiornis , Xiaotingia , troodontids and some basal dromaeosaurids [2] , [3] . The teeth of Eosinopteryx are unserrated and sharp in contrast to the bulbous teeth of Xiaotingia [3] . As characteristic of troodontids [5] , the premaxillary and the dentary teeth in the symphyseal region are more closely packed than are the teeth in the posterior part of the dentary. 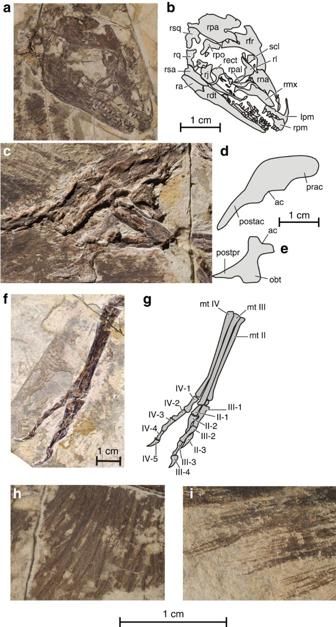Figure 2: Selected skeletal elements and associated feathers ofEosipnopteryx brevipennaYFGP-T5197. (a) Photograph of skull and mandible in right lateral view. (b) Line drawing of skull and mandible in right lateral view. (c) Photograph of pelvis in right lateral view. (d) Line drawing of right ilium in lateral view. (e) Line drawing of right ischium in lateral view. (f) Photograph of right metatarsus and pes. (g) Line drawing of right metatarsus and pes. (h) Detail of secondary remiges. (i) Detail of plumulaceous feathers under the middle part of the tail. ac, acetabulum; lpm, left premaxilla; mt, metatarsal; obt, obturator process; postpr, posterodistal process; prac, preacetabular process; ra, right angular; rdt, right dentary; rect, right ectopterygoid; rfr, right frontal; rj, right jugal; rl, right lacrimal; rmx, right maxilla; rna, right nasal; rpa, right parietal; rpal, right palatine; rpm, right premaxilla; rpo, right postorbital; rq, right quadrate; rsq, right squamosal; rsa, right surangular; scl, scleral plate. Figure 2: Selected skeletal elements and associated feathers of Eosipnopteryx brevipenna YFGP-T5197. ( a ) Photograph of skull and mandible in right lateral view. ( b ) Line drawing of skull and mandible in right lateral view. ( c ) Photograph of pelvis in right lateral view. ( d ) Line drawing of right ilium in lateral view. ( e ) Line drawing of right ischium in lateral view. ( f ) Photograph of right metatarsus and pes. ( g ) Line drawing of right metatarsus and pes. ( h ) Detail of secondary remiges. ( i ) Detail of plumulaceous feathers under the middle part of the tail. ac, acetabulum; lpm, left premaxilla; mt, metatarsal; obt, obturator process; postpr, posterodistal process; prac, preacetabular process; ra, right angular; rdt, right dentary; rect, right ectopterygoid; rfr, right frontal; rj, right jugal; rl, right lacrimal; rmx, right maxilla; rna, right nasal; rpa, right parietal; rpal, right palatine; rpm, right premaxilla; rpo, right postorbital; rq, right quadrate; rsq, right squamosal; rsa, right surangular; scl, scleral plate. Full size image There are seven postaxial cervical vertebrae in YFGP-T5197. The cervical ribs are as long as their corresponding centra, contrasting with the shorter cervical ribs seen in Troodon formosus [5] and the much longer ones of Archaeopteryx [6] . The trunk is about 32% the length of the hindlimb, as in Anchiornis [2] and Mei [7] . The middle and posterior dorsals are proportionally elongate as in Anchiornis , dromaeosaurids and Archaeopteryx [8] . As in the latter, Anchiornis and basal deinonychosaurs, the dorsal centra do not have distinct pneumatic foramina just shallow depressions on their lateral surfaces [3] . Numerous, very slender, abdominal ribs are preserved in YFGP-T5197, as in Archaeopteryx [6] , dromaeosaurids [9] , the basal pygostylian bird Confuciusornis [10] and many enantiornithines (for example, Sinornis ). The tail of Eosinopteryx is particularly short, 2.7 times the length of the femur (contrasting with 3.2 in Mei [7] and 3.9 in the Eichstätt Archaeopteryx [6] ), and only composed of 20 caudal vertebrae (contrasting with 21–23 in Archaeopteryx [6] , ca. 30 in Anchiornis [1] and 24–26 in Microraptor [11] ). The anterior caudals are proportionally short, their transverse processes longer than corresponding centra and particularly narrow. Neural spines are developed only on the anteriormost third or fourth caudals. As in Anchiornis and Archaeopteryx [2] , [3] , the middle and posterior caudal vertebrae each bear a distinct groove on the lateral surface near the junction of the centrum and neural arch. The chevrons are reduced to small rod-like elements and are only present below the proximal eighth or ninth caudal centra, contrasting with the larger hook-like proximal chevrons of Anchiornis [1] and with the vertically oriented rectangular proximal chevrons of Archaeopteryx [6] . The subrectangular coracoid of Eosinopteryx bears a distinct subglenoid fossa and has a wider proximal end than Xiaotingia [3] ( Supplementary Fig. S1 ). The scapula (scapula/femur=0.49) is proportionally much shorter than in Anchiornis (0.68). The forelimb of this small paravian (0.73 times hindlimb length) is slightly shorter than that of Anchiornis (0.8) (ref. 2 ) and Archaeopteryx (0.9–1.0) (ref. 6 ) but is much longer than Mei (0.5) (ref. 7). The humerus of Eosinopteryx is also shorter (0.8 times) than its femur; the humerus is slightly longer than the femur in Anchiornis , distinctly longer (1.1–1.2) (ref. 6) in Archaeopteryx , and is only half the femur length in Mei . As in Anchiornis , the radius and ulna of Eosinopteryx are straight with only a narrow gap between them. The manus is slightly longer than the femur (manus/femur=1.2), contrasting with the short hand of Mei (0.8) (ref. 7) and with the proportionally more elongate hands of Anchiornis (1.55) (ref. 2) and Archaeopteryx (1.4–1.6) (ref. 6). Metacarpal II is about one third the length of metacarpal III; in contrast to Xiaotingia [3] , metacarpal IV is shorter and is much more slender than metacarpal III ( Supplementary Fig. S2 ). The phalangeal portion of the manus is also proportionally shorter, relative to the metacarpus, than in Xiaotingia [3] . As in Anchiornis [2] , the long manual phalanx II-1 of Eosinopteryx is as robust as the radius; this element is much more gracile in Sinornithoides [12] and Archaeopteryx [6] . Contrasting with Xiaotingia [3] , phalanx III-2 is shorter than metacarpal III, whereas the manual unguals of Eosinopteryx , sheathed by long keratinous claws, are less curved than in Archaeopteryx [6] , Anchiornis [1] and Xiaotingia [3] . The ilium of Eosinopteryx is characterized by a long, low and distally tapering postacetabular process, with a ratio ‘length/height at mid-length’ of 5 ( Fig. 2 ). The ischium is particularly short, about 28% the femur length. With its distally displaced obturator process and its long and pointed posterodistal process, this element closely resembles that of Anchiornis [1] , [2] ( Fig. 2 ). The tibiotarsus of Eosinopteryx (1.4 × femur length) is proportionally shorter than Anchiornis (1.60), whereas pes (metatarsus+phalanges) proportions (1.3 × femur length) are similar to those of Mei [7] and shorter than Anchiornis (1.56) (ref. 2). The proximal end of metatarsal III is transversely compressed, suggesting a subarctometatarsalian condition. Pedal digit I lies on the medioplantar side of metatarsal II ( Fig. 2 ), as in Archaeopteryx [6] , [13] , [14] , but contrasts with the position of pedal digit I in Anchiornis, which is medial to metatarsal II [1] . The phalanges of pedal toes II, III and IV decrease gradually in length proximodistally, as in Archaeopteryx and terrestrial cursorial birds [15] . The pedal unguals of Eosinopteryx are much shorter than those of Archaeopteryx [6] , Anchiornis [1] , [2] , troodontids [5] and dromaeosaurids [9] , even shorter than the corresponding penultimate phalanges. As in Anchiornis [2] , the longest remiges of Eosinopteryx are at least 150% the length of the humerus ( Fig. 2 ) and are symmetrical on the forelimbs. Long, densely packed and symmetrical pennaceous feathers are present along the posterior part of the thigh and crus, consistent in distribution with the tetrapterygian condition of several other basal paravian taxa [2] , [16] . However, careful preparation shows that feathers were absent from the metatarsus and pes of YFGP-T5197. Feathers covering other regions of the body (head, neck, thorax, back and tail) are plumulaceous and ‘rachis-like’ structures described on the plumulaceous feathers at the base of the tail and on the neck in Mei [7] are absent in Eosinopteryx . The feathers on the tail are short, <20 mm long; all are plumulaceous, composed of a bundle of filaments that are joined together proximally and remain nearly parallel as they pass distally ( Fig. 2 ). Pennaceous rectrices are absent. Preliminary phylogenetic analysis places E. brevipenna sister to Anchiornis huxleyi at the base of Troodontidae ( Fig. 3 ) (subject to change in subsequent analyses; see Supplementary Methods for details). Both taxa share a dorsally curved ilium shaft, a pubis moderately oriented posteriorly and a straight ulna that is not bowed away from the humerus. Archaeopteryx and Wellnhoferia form an unresolved polytomy at the base of Deinonychosauria in the strict consensus tree, supporting the hypothesis that Archaeopteryx is a deinonychosaurian theropod instead of a primitive bird [3] ( Fig. 3 ). Note, however, that this phylogeny remains only weakly supported presumably due to the numerous homoplasies widely distributed across coelurosaurian phylogeny [3] , [17] ( Supplementary Fig. S3 ). 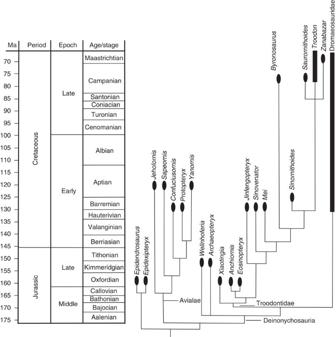Figure 3: Phylogeny of Paraves. Time-calibrated strict consensus tree of the 10 most-parsimonious trees. Tree length=1,386; consistency index (CI) excluding uninformative characters=0.3; retention index (RI)=0.7. We added four feather-related characters to the original matrix3but these do not influence the topology of the strict consensus tree. Character 375: remiges on the forelimb absent (0) or present (1); character 376: pennaceous feathers on the tibia absent (0) or present (1); character 377: feathers on metatarsus and pes absent (0) or present (1); character 378: rectrices absent (0) or present (1). Figure 3: Phylogeny of Paraves. Time-calibrated strict consensus tree of the 10 most-parsimonious trees. Tree length=1,386; consistency index (CI) excluding uninformative characters=0.3; retention index (RI)=0.7. We added four feather-related characters to the original matrix [3] but these do not influence the topology of the strict consensus tree. Character 375: remiges on the forelimb absent (0) or present (1); character 376: pennaceous feathers on the tibia absent (0) or present (1); character 377: feathers on metatarsus and pes absent (0) or present (1); character 378: rectrices absent (0) or present (1). Full size image The almost complete plumage of Eosinopteryx is less developed than that of other known Middle-Late Jurassic deinonychosaurians. The complete absence of rectrices on the tail cannot be explained by taphonomic factors (that is, more fragile plumulaeous feathers are well preserved along the whole length of the tail) and does not reflect a basal phylogenetic position for Eosinopteryx among paravians, because long rectrices are now known to occur in at least one basal member of each of the five major known lineages in this region of the theropod tree, including basal avialans, the basal deinonychosaurians Archaeopteryx and Wellnhoferia [6] , the basal troodontid Anchiornis [18] , the scansoriopterygid Epidexipteryx [19] and the basal dromaeosaurid Microraptor [20] . The secondary loss of rectrices is regarded here as an unambiguous autapomorphy for E. brevipenna ( Fig. 4 ). Pennaceous rectrices attached to the tibia were also a relatively ubiquotous adaptation among maniraptorans, present in Eosinopteryx , Anchiornis [2] , Xiaotingia [3] , Microraptor [15] , Pedopenna [21] , Archaeopteryx and Wellnhoferia [6] ; this character is regarded here as an unambiguous synapomorphy for Deinonychosauria ( Fig. 4 ). 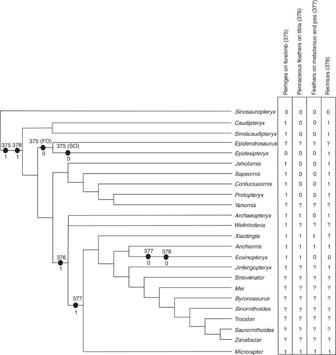Figure 4: Mapping of feather characters onto a simplified strict consensus tree. FO, fast optimization. SO, slow optimization. If not denoted, mapping is unambiguous. Figure 4: Mapping of feather characters onto a simplified strict consensus tree. FO, fast optimization. SO, slow optimization. If not denoted, mapping is unambiguous. Full size image In this phylogeny, the presence of long feathers on the metatarsus and pes, observed in Anchiornis [2] , Xiaotingia [3] and Microraptor [16] , is regarded as an unambiguous synapomorphy for the clade Troodontidae+Dromaeosauridae, and their secondary loss an unambiguous autapomorphy for Eosinopteryx ( Fig. 4 ). It cannot be totally excluded that the absence of pennaceous feathers on the metatarsus and pes of Eosinopteryx is a preservational artefact, because other integumental features (for example, scales or scutes) are not preserved at the same location. However, scutes and scales on the lower leg have never been identified in any feathered dinosaur or Mesozoic bird described to date. Despite its small size, the holotype of Eosinopteryx had reached a late ontogenetic stage (subadult or adult): neurocentral sutures are closed on all exposed vertebrae ( Supplementary Fig. S4 ) and the suture between the astragalus–calcaneum complex and the tibia cannot be discerned ( Supplementary Fig. S5 ). Ontogenetic stage, therefore, also cannot account for reduced plumage, although temporary disappearance of rectrices and pennaceous feathers on the metatarsus and pes might be explained by a seasonal moult. It is parsimonious that the plumage differences of Eosinopteryx can be explained by its mode-of-life. With a shorter humerus and manus and a reduced plumage, Eosinopteryx had a much shorter wing span than other feathered paravians including Archaeopteryx , Wellnhoferia and Anchiornis . The straight and closely aligned ulna-radius of Eosinopteryx also means that pronation/supination of the manus with respect to the upper arm would have been limited; combined with the absence of a bony sternum and weakly developed proximal humerus, these attributes suggest that Eosinopteryx had little or no ability to oscillate the arms to produce a wing beat. The phalanges of the third toe of Eosinopteryx decrease proximodistally and its ungual phalanges are not very recurved and particularly short, suggesting a ground dwelling, ‘cursorial’ mode-of-life as in many living birds [15] . Reduced plumage on the tail and lower legs would have facilitated this ecology and allowed Eosinopteryx to run easily. This new specimen also shows that the plumage of paravian theropods was already diversified by the Late Jurassic and already had different functions: insulation, flight and visual display [19] , [20] . Although Anchiornis and Eosinopteryx are clearly similar from osteological and phylogenetic points-of-view, their plumage shows that they were adapted to different ecological niches and implies a much more complex picture in terms of the origin of flight than often supposed. Indeed, it is likely that the diversification of integumental structures facilitated the sympatry of numerous closely related paravian theropods in the Late Jurassic Tiaojishan Formation and later in the Early Cretaceous Jehol Group. Origin and authenticity of the specimen As it is the case for most of the paravian specimens known from western Liaoning Province, the holotype and only known specimen of E. brevipenna was acquired by the Yizhou Fossil & Geology Park from a Chinese fossil dealer, according to whom the specimen was collected at the Yaolugou locality (Jianchang county, western Liaoning, China), not far from Daxishan village where A. huxlei specimen LPM (Liaoning Paleontological Museum)-B00169 was discovered [2] . The Tiaojishan formation is widely exposed in this area [22] , though it also has limited outcrops of the Early Cretaceous Yixian Formation [23] . The E. brevipenna specimen is preserved in a shale slab, the sedimentary structures of which closely resemble those of the specimens of A. huxlei and Xiaotingia zhengi also described from the Tiaojishan Formation; it is in fact extremely difficult to distinguish between Tiaojishan and Yixian shale slabs on the basis of macro-sedimentary features. It is, therefore, necessary to study in detail the micro-sedimentary structures and the pollen assemblages within the shale slabs to certify the age of the specimen, as it is also the case for the A. huxlei and Xioatingia zhengi specimens described so far [3] . The specimen was only partially prepared when it was sold by the Chinese dealer. Careful preparation by the Yizhou Fossil & Geology Park staff and by authors of this paper (FE and PG) did not reveal any trace of forgery, and the probability that the specimen is a composite is accordingly low. Age of the Tiaojishan Formation The Tiaojishan Formation crops out in the West Liaoning Province and is equivalent to the Lanqi Formation of North Hebei Province [24] . The reason for the abundance of excellently preserved fossils is the presence of interbedded tuffs originating from recurrent volcanic events [25] . In western Liaoning, the Tiaojishan Formation is 130–970 m thick [25] and is composed of different types of rocks, including basalts, andesites, rhyolites, tuffs, tuffaceous sandstones and conglomerates [24] , [25] . Because of the complicated stratigraphic pattern in the Tiaojishan Formation, accurate dating of the formation is particularly difficult [24] . Ages between 165±1.2 Ma and 153±2 Ma were obtained by SHRIMP U-Th-Pb analysis of samples from the Tiaojishan (=Lanqi) Formation [26] . Zhang et al . [24] concluded that the upper boundary of the Tiaojishan (=Lanqi) formation dates between 156 and 153 Ma. Chang et al . [25] obtained Ar-Ar ages of 160.7±0.4 Ma and 158.7±0.6 Ma for the basal Lanqi Formation in North Hebei Province. These results indicate that the age of the Tiaojishan Formation is between the Callovian (Middle Jurassic) and the Kimmeridgian (Late Jurassic) [27] . Nomenclatural acts This published work and the nomenclatural acts it contains have been registered in ZooBank, the proposed online registration system for the International Code of Zoological Nomenclature. The ZooBank LSIDs (Life Science Identifiers) can be resolved and the associated information viewed through any standard web browser by appending the LSID to the prefix ‘ http://zoobank.org/ ’. The LSIDs for this publication are: urn:lsid:zoobank.org:act:068F0446-C80D-4F90-837C-921AB291880F; urn:lsid:zoobank.org:pub:11EEC3B6-1BF7-4DDE-872F-C84DE2CBBA20. How to cite this article: Godefroit, P. et al . Reduced plumage and flight ability of a new Jurassic paravian theropod from China. Nat. Commun. 4:1394 doi: 10.1038/ncomms2389 (2013).